Disruption of TBP-2 ameliorates insulin sensitivity and secretion without affecting obesity Type 2 diabetes mellitus (T2DM) is characterized by defects in both insulin sensitivity and glucose-stimulated insulin secretion (GSIS) and is often accompanied by obesity. In this study, we show that disruption of thioredoxin binding protein-2 (TBP-2, also called Txnip) in obese mice (ob/ob) dramatically improves hyperglycaemia and glucose intolerance, without affecting obesity or adipocytokine concentrations. TBP-2-deficient ob/ob mice exhibited enhanced insulin sensitivity with activated insulin receptor substrate-1/Akt signalling in skeletal muscle and GSIS in islets compared with ob/ob mice. The elevation of uncoupling protein-2 (UCP-2) expression in ob/ob islets was downregulated by TBP-2 deficiency. TBP-2 overexpression suppressed glucose-induced adenosine triphosphate production, Ca 2+ influx and GSIS. In β-cells, TBP-2 enhanced the expression level and transcriptional activity of UCP-2 by recruitment of peroxisome proliferator-activated receptor-γ co-activator-1α to the UCP-2 promoter. Thus, TBP-2 is a key regulatory molecule of both insulin sensitivity and GSIS in diabetes, raising the possibility that inhibition of TBP-2 may be a novel therapeutic approach for T2DM. Regulation of glucose homeostasis is critical to life in mammals and is largely maintained by pancreatic β-cells, which secrete insulin in response to increased concentrations of glucose, and is also maintained by the glucose uptake response to insulin in peripheral tissues. Obesity disrupts glucose homeostasis and leads to diseases such as type 2 diabetes (T2DM), which is characterized by aggravated insulin sensitivity and insulin secretion [1] , [2] , [3] , [4] , [5] . Thioredoxin binding protein-2 (TBP-2), also known as thioredoxin interacting protein (Txnip) [6] and vitamin-D3 upregulated protein-1 (VDUP1) [7] , has been identified as a negative regulator of thioredoxin and is mainly localized in the nucleus [8] , [9] . TBP-2 is a member of the α-arrestin protein family, and contains two characteristic arrestin-like domains and two PPxY sequences, which is a known binding motif for WW domain containing proteins [10] , [11] , [12] . Evidence is growing that TBP-2 has an important role in a wide variety of biological functions, such as the regulation of cell death, cell growth, cell differentiation, immune responses and energy metabolism [13] , [14] , [15] , [16] , [17] , [18] , [19] , [20] , [21] , [22] . As our group and others have shown that TBP-2-deficient mice or mice carrying the TBP-2 nonsense mutation (HcB-19) have increased insulin sensitivity [16] , [20] , [23] and insulin secretion [16] , [18] , we hypothesized that TBP-2 is involved in defects of insulin sensitivity and secretion in diabetes. In this study, to address the physiological and molecular role of TBP-2 in diabetes, we generated a TBP-2-deficient diabetic mice model (ob/ob·TBP-2−/−). Remarkably, these mice displayed improved glucose intolerance due to enhanced muscle insulin sensitivity associated with the insulin receptor substrate-1 (IRS-1)/Akt pathway and glucose-stimulated insulin secretion (GSIS) in spite of obesity. The augmented insulin secretion was due to the elevation of glucose-induced adenosine triphosphate (ATP) production with suppression of mitochondrial uncoupling protein-2 (UCP-2) expression. UCP-2 is known as a negative regulator of GSIS in diabetes [24] . We showed that TBP-2 regulates insulin secretion mainly through UCP-2 transcriptional activation in β-cell lines. We further investigated mechanisms for TBP-2 regulation of UCP-2 transcription and analysed interacting proteins for TBP-2 in β-cells. The current results provide a novel mechanism for elucidating the pathogenesis of diabetes. Disruption of TBP-2 in ob/ob mice improves hyperglycaemia Subsequent to a report that TBP-2 expression is elevated in skeletal muscle of patients with impaired glucose tolerance or T2DM [19] , we examined the expression levels of TBP-2 mRNA in the tissues of leptin-deficient (ob/ob) mice; a genetic animal model of human obesity and T2DM. Expression levels of TBP-2 were increased in the heart, skeletal muscle, white adipose tissue, kidney and pancreatic islets, but were not significantly changed in the liver of ob/ob mice compared with wild-type (WT) lean mice ( Fig. 1a ). To determine how TBP-2 is involved in the development of diabetic phenotypes in obese mice, we next studied the effect of endogenous TBP-2 in ob/ob mice by generating TBP-2-deficient ob/ob mice (ob/ob·TBP-2−/−) ( Fig. 1b ). Ob/ob·TBP-2−/− mice did not show any significant change in food intake, but showed reduced water intake compared with that of ob/ob mice ( Fig. 1c,d ). Surprisingly, although body weight was higher in male and as high in female ob/ob·TBP-2−/− mice compared with that in ob/ob mice ( Fig. 1e,g ), TBP-2 deficiency markedly improved hyperglycaemia and urinary glucose excretion both in male and female ob/ob mice ( Fig. 1f,h,i ). Furthermore, glucose tolerance tests revealed significant amelioration of glucose metabolism in ob/ob·TBP-2−/− mice ( Fig. 1j,k ), consistent with insulin tolerance tests (ITTs) in which insulin sensitivity significantly increased in ob/ob·TBP-2−/− mice compared with that in ob/ob mice ( Fig. 1l,m ). These results suggest that disruption of TBP-2 in ob/ob mice improves glucose tolerance and insulin sensitivity. 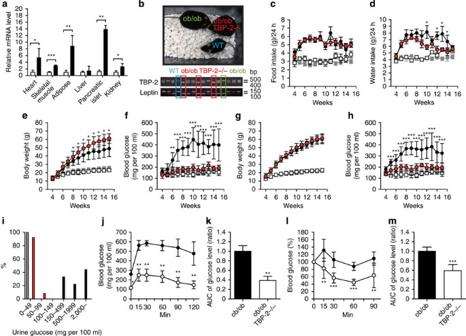Figure 1: Disruption of TBP-2 in ob/ob mice improves hyperglycaemia and glucose intolerance without affecting obesity. (a) Quantitative RT–PCR ofTBP-2expression in the heart, skeletal muscle, white adipose, liver, pancreatic islet and kidney of WT (open bar, lean,n=3) and ob/ob mice (closed bar,n=3). (b) Generation of the ob/ob·TBP-2−/− mice. Male food intake (c), male water intake (d), male body weight (e), male blood glucose in fedad lib(f), female body weight (g), female blood glucose in fedad lib(h) were assessed,N≥6. WT, grey rectangles; TBP-2−/−, white rectangles; ob/ob, black circles; ob/ob·TBP-2−/−, red circles. (i) Urine glucose (mg per 100 ml) of males and females. WT (grey bar;n=11), ob/ob (black bar;n=9), ob/ob·TBP-2−/− (red bar;n=11). (j,k) Intraperitoneal glucose tolerance test (IPGTT). Following an overnight fast, mice were injected with 0.5g kg−1glucose, IP (time 0). Blood glucose values (j) and area under the curve (AUC) levels (k) were assessed before and at 15, 30, 60 and 120 min into the IPGTT. ob/ob (black circle,n=5), ob/ob·TBP-2−/− (white circle,n=6). (l,m) IP insulin tolerance test (IPITT). Following a 6 h fast, mice were injected with 1 U/kg of insulin, i.p. (time 0). Blood glucose value (l) and AUC levels (m) were assessed before and at 15, 30, 60 and 90 min into the IPITT. ob/ob (black circle,n=5), ob/ob·TBP-2−/− (white circle,n=6). Data are presented as mean±s.d. *P<0.05, **P<0.01, ***P<0.001, versus control (t-test). Figure 1: Disruption of TBP-2 in ob/ob mice improves hyperglycaemia and glucose intolerance without affecting obesity. ( a ) Quantitative RT–PCR of TBP-2 expression in the heart, skeletal muscle, white adipose, liver, pancreatic islet and kidney of WT (open bar, lean, n =3) and ob/ob mice (closed bar, n =3). ( b ) Generation of the ob/ob·TBP-2−/− mice. Male food intake ( c ), male water intake ( d ), male body weight ( e ), male blood glucose in fed ad lib ( f ), female body weight ( g ), female blood glucose in fed ad lib ( h ) were assessed, N ≥6. WT, grey rectangles; TBP-2−/−, white rectangles; ob/ob, black circles; ob/ob·TBP-2−/−, red circles. ( i ) Urine glucose (mg per 100 ml) of males and females. WT (grey bar; n =11), ob/ob (black bar; n =9), ob/ob·TBP-2−/− (red bar; n =11). ( j , k ) Intraperitoneal glucose tolerance test (IPGTT). Following an overnight fast, mice were injected with 0.5g kg −1 glucose, IP (time 0). Blood glucose values ( j ) and area under the curve (AUC) levels ( k ) were assessed before and at 15, 30, 60 and 120 min into the IPGTT. ob/ob (black circle, n =5), ob/ob·TBP-2−/− (white circle, n =6). ( l , m ) IP insulin tolerance test (IPITT). Following a 6 h fast, mice were injected with 1 U/kg of insulin, i.p. (time 0). Blood glucose value ( l ) and AUC levels ( m ) were assessed before and at 15, 30, 60 and 90 min into the IPITT. ob/ob (black circle, n =5), ob/ob·TBP-2−/− (white circle, n =6). Data are presented as mean±s.d. * P <0.05, ** P <0.01, *** P <0.001, versus control ( t -test). Full size image TBP-2 deficiency ameliorates insulin resistance As altered production of adipocytokines accompanied with obesity is implicated in insulin resistance and glucose intolerance [2] , [25] , body fat composition, serum monocyte chemotactic protein-1 (MCP-1), adiponectin and metabolic parameters of ob/ob·TBP-2−/− mice were measured. In ob/ob·TBP-2−/− mice, body fat and serum levels of fatty acids, MCP-1 and lipids increased and serum adiponectin decreased compared with those in WT and/or ob/ob mice ( Fig. 2a–i and Supplementary Table S1 ). TBP-2 deficiency in ob/ob mice did not improve adipose size, and TBP-2−/− mice showed increased adipose size compared with that in WT mice ( Fig. 2j ). These results show that TBP-2 deficiency improves insulin sensitivity without amelioration of overeating, obesity and adipocyte dysfunction. 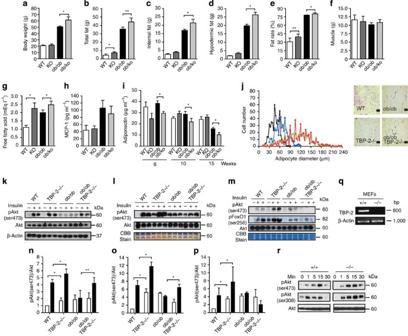Figure 2: TBP-2 deficiency ameliorates insulin resistance and increase Akt signalling. (a–f) Fat and muscle content. Body weight (a), total fat (b), internal fat (c), hypodermic fat (d), fat rate (e), muscle (f) in male WT (WT), TBP-2−/− (KO), ob/ob (ob/ob) and ob/ob·TBP-2−/− (ob/ko) mice calculated from computed tomography scan data are shown for 15 weeks aged mice,N≥4. (g,h) Serum physiological parameters. Free fatty acid (g) and MCP-1 (h) were measured in 15 weeks aged mice,N≥7. (i) Blood adiponectin concentration was measured in 6, 10 and 15 weeks aged mice,n=≥5. (j) Distribution of adipocyte size in white adipose from 10 weeks aged WT (black closed rectangle), TBP-2−/− (blue open rectangle), ob/ob (green closed circle) and ob/ob·TBP-2−/− (red open circle) mice (left panel). The right panel shows histological analyses of haematoxylin and eosin (HE)-stained white adipose sections in these mice. Scale bar indicates 100 μm. (k–m) Immuno blotting (IB) analyses of ser473-phospholylated Akt (pAkt), ser256-phospholylated FoxO1 (pFoxO1) and total Akt in response to insulin (2 U kg−1) in skeletal muscle (k), heart (l) and liver (m). Densitometric quantification of pAkt/Akt ratios in skeletal muscle (n), heart (o) and liver (p). Open and closed bar represents without or with insulin stimulation, respectively. (q) Loss of endogenous TBP-2 mRNA in MEFs. (r) IB analyses. TBP-2 deficiency enhances insulin/Akt signalling in primary MEFs. MEFs were serum starved for 12 h and then stimulated with insulin (100 nM) for different times. Data are presented as mean±s.d. *P< 0.05, **P< 0.01, versus control (t-test). Figure 2: TBP-2 deficiency ameliorates insulin resistance and increase Akt signalling. ( a – f ) Fat and muscle content. Body weight ( a ), total fat ( b ), internal fat ( c ), hypodermic fat ( d ), fat rate ( e ), muscle ( f ) in male WT (WT), TBP-2−/− (KO), ob/ob (ob/ob) and ob/ob·TBP-2−/− (ob/ko) mice calculated from computed tomography scan data are shown for 15 weeks aged mice, N ≥4. ( g , h ) Serum physiological parameters. Free fatty acid ( g ) and MCP-1 ( h ) were measured in 15 weeks aged mice, N ≥7. ( i ) Blood adiponectin concentration was measured in 6, 10 and 15 weeks aged mice, n =≥5. ( j ) Distribution of adipocyte size in white adipose from 10 weeks aged WT (black closed rectangle), TBP-2−/− (blue open rectangle), ob/ob (green closed circle) and ob/ob·TBP-2−/− (red open circle) mice (left panel). The right panel shows histological analyses of haematoxylin and eosin (HE)-stained white adipose sections in these mice. Scale bar indicates 100 μm. ( k – m ) Immuno blotting (IB) analyses of ser473-phospholylated Akt (pAkt), ser256-phospholylated FoxO1 (pFoxO1) and total Akt in response to insulin (2 U kg −1 ) in skeletal muscle ( k ), heart ( l ) and liver ( m ). Densitometric quantification of pAkt/Akt ratios in skeletal muscle ( n ), heart ( o ) and liver ( p ). Open and closed bar represents without or with insulin stimulation, respectively. ( q ) Loss of endogenous TBP-2 mRNA in MEFs. ( r ) IB analyses. TBP-2 deficiency enhances insulin/Akt signalling in primary MEFs. MEFs were serum starved for 12 h and then stimulated with insulin (100 nM) for different times. Data are presented as mean±s.d. * P < 0.05, ** P < 0.01, versus control ( t -test). Full size image As insulin resistance is derived from defects in insulin signalling in peripheral tissues, [1] and insulin/Akt signalling regulates many of the metabolic actions of insulin [1] , we investigated phosphorylation of Akt in these mice. Akt phosphorylation levels in both basal- and insulin-stimulated states were upregulated in skeletal muscle, heart and liver of TBP-2−/− mice compared with those in WT mice ( Fig. 2k–p ). In addition, TBP-2 deficiency enhanced Akt phosphorylation levels in response to insulin in mouse embryonic fibroblasts (MEFs) ( Fig. 2q,r ), suggesting that TBP-2 deficiency enhances insulin/Akt signalling. Although ob/ob mice showed suppression of Akt phosphorylation in response to insulin in skeletal muscle, heart and liver, compared with those in WT mice without affecting the concentration of total Akt protein, TBP-2 deficiency in ob/ob mice restored the suppression of Akt phosphorylation in skeletal muscle and heart, but not liver ( Fig. 2k–p ). The phosphorylation of FoxO1, an Akt downstream signalling molecule, was also not enhanced in the liver of ob/ob·TBP-2−/− mice. Severe lipid accumulation occurred in the liver both in ob/ob and ob/ob·TBP-2−/− mice ( Supplementary Fig. S1a,b ). Thus, the amelioration of insulin sensitivity by TBP-2 deficiency in ob/ob mice seems to be due to activation of insulin/Akt signalling in skeletal muscle. TBP-2 deficiency enhances IRS-1 expression in skeletal muscle We performed microarray analyses (data deposited in GEO, accession number GSE24851 ) of the skeletal muscle in WT, TBP-2−/−, ob/ob, ob/ob·TBP-2−/− mice to investigate how TBP-2 regulates Akt signalling and insulin sensitivity. We found that several insulin signalling-related genes, such as Igf1, Igf2bp2, Igfbp4, Irs-1(IRS-1), Pik3r1 and Pik3r5 , were upregulated by TBP-2 deficiency both in WT and ob/ob background mice ( Supplementary Table S2 ). The upregulation was confirmed by real-time reverse transcription (RT)–PCR analyses ( Fig. 3a ). IRS-1 gene expression was downregulated in skeletal muscle of ob/ob mice ( Fig. 3a ) or T2DM patients [26] . We focused on IRS-1, as IRS-1 is one of the key molecules for insulin signalling and is an upstream molecule of Akt in skeletal muscle [27] . IRS-1 protein levels were downregulated in ob/ob mice, whereas IRS-1 protein levels and phosphorylation of Akt were upregulated by TBP-2 deficiency in skeletal muscle of WT and ob/ob background mice ( Fig. 3b ). Thus, TBP-2 regulates the expression of molecules involved in insulin signalling, which may enhance insulin sensitivity in skeletal muscle. Gene expressions of peroxisome proliferator-activated receptor (PPAR) signalling were also enhanced by TBP-2 deficiency in skeletal muscle ( Supplementary Fig.S2 ). 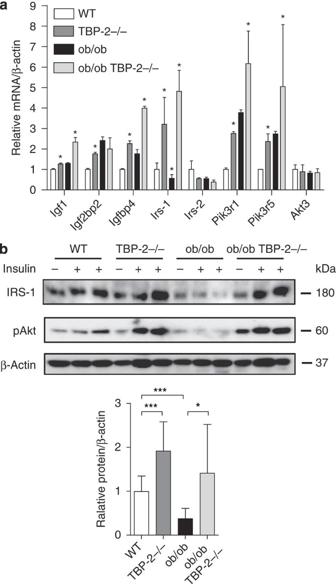Figure 3: Insulin signalling-related genes are upregulated by TBP-2 deficiency in skeletal muscle. The expression of insulin signal-related genes from the skeletal muscle of 10 weeks aged WT (white bar), TBP-2−/− (dark grey bar), ob/ob (black bar) and ob/ob·TBP-2−/− (light grey bar) mice. (a) Real-time PCR analyses were performed. Asterisk indicates *P<0.05 ;WT versus TBP-2−/−, WT versus ob/ob, ob/ob versus ob/ob·TBP-2−/−. (b) Immuno blotting (IB) analyses,nper group 3–5 each. Two U kg−1insulin (+) or saline (−) was injected. Densitometric quantification of IRS-1/β-actin is shown in the bar graph. Data are presented as mean±s.d. *P<0.05, ***P<0.001, versus control (t-test). Figure 3: Insulin signalling-related genes are upregulated by TBP-2 deficiency in skeletal muscle. The expression of insulin signal-related genes from the skeletal muscle of 10 weeks aged WT (white bar), TBP-2−/− (dark grey bar), ob/ob (black bar) and ob/ob·TBP-2−/− (light grey bar) mice. ( a ) Real-time PCR analyses were performed. Asterisk indicates * P <0.05 ;WT versus TBP-2−/−, WT versus ob/ob, ob/ob versus ob/ob·TBP-2−/−. ( b ) Immuno blotting (IB) analyses, n per group 3–5 each. Two U kg −1 insulin (+) or saline (−) was injected. Densitometric quantification of IRS-1/β-actin is shown in the bar graph. Data are presented as mean±s.d. * P <0.05, *** P <0.001, versus control ( t -test). Full size image TBP-2 deficiency improved impairment of insulin secretion TBP-2−/− mice and HcB-19 mice show enhanced insulin secretion in vivo [16] , [18] . Although obesity usually leads to insulin resistance, only a subset of obese- and insulin-resistant individuals progress to T2DM. In ob/ob mice and humans, the determinant factor for declining glucose tolerance is a progressive decrease in GSIS [3] . Of note, ob/ob mice showed elevated blood glucose with an increase in body weight after ages 5 or 6 weeks, whereas TBP-2-deficient ob/ob mice did not show elevation of blood glucose, in spite of similar increases in body weight. In addition, although blood glucose levels were lower in ob/ob·TBP-2−/− mice, compared with those in ob/ob mice, serum insulin levels in ob/ob·TBP-2−/− mice were as high as those in ob/ob mice at ages 11 and 14 weeks in both males and females ( Fig. 4a,b ). Although we observed no significant change in islet mass between ob/ob·TBP-2−/− mice and ob/ob mice, as well as between TBP-2−/− and WT mice ( Fig. 4c,d ), serum insulin levels after glucose loads in vivo were enhanced in ob/ob·TBP-2−/− mice compared with those in ob/ob mice ( Fig. 4e ). To evaluate the effect of TBP-2 deficiency on insulin secretion ex vivo , pancreatic islets were isolated from WT, TBP-2−/−, ob/ob and ob/ob·TBP-2−/− mice. TBP-2 deficiency enhanced GSIS in both WT and ob/ob mice ( Fig. 4f,g ). Insulin secretion from ob/ob islets in response to high glucose was blunted, and was improved by TBP-2 deficiency ( Fig. 4g,h ). These results suggest that TBP-2 deficiency improves impairment of GSIS from islets, which contributes to improvement of glucose intolerance in ob/ob mice. As glucose metabolism generates ATP as a signal to enhance insulin secretion [28] , we further determined ATP content of islets in these mice. Under a high (16.7 mM) glucose condition, TBP-2 deficiency enhanced ATP content in both WT and ob/ob islets ( Fig. 4i,j ). WT islets showed a significant increase in ATP production with increased glucose concentrations ( Fig. 4i ). In ob/ob islets, increases in ATP content with increasing glucose levels were not as marked ( Fig. 4j,k ), as in TBP-2 deficiency where the ratio of ATP content at high glucose (16.7 mM) relative to basal glucose (2.8 mM) was significantly increased ( Fig. 4k ). Regulation of mitochondrial ATP production has a central role in insulin secretion from pancreatic β-cells [4] and the reduction of mitochondrial ATP production parallels abnormal mitochondrial structure, including swelling and alteration in volume density and cristae structure [29] , which is often observed in diabetes [5] , [30] . We then studied the morphology of mitochondria in WT, TBP-2−/−, ob/ob and ob/ob·TBP-2−/− β-cells using electron microscopy. Morphological apoptotic processes, including condensation of chromatin around the nuclear membrane and swelling of the cytoplasm and a decrease in the number of insulin granules in β-cells, were not observed in ob/ob and ob/ob·TBP-2−/− mice at 10 weeks ages ( Supplementary Fig. S3a,b ). However, the abnormal mitochondrial morphological changes, such as swelling associated with an increased number of disarrayed or disappeared cristae and a reduced electron density of the matrix, were observed in ob/ob mice, whereas the abnormalities were improved in ob/ob·TBP-2−/− mice ( Fig. 4l ). These results showed that mitochondrial morphological changes and metabolic dysfunctions in β-cells are improved by TBP-2 deficiency in ob/ob mice. 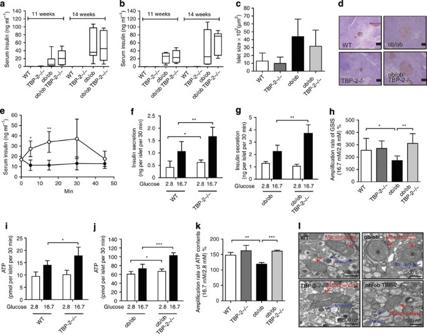Figure 4: Impairment of glucose-stimulated insulin secretion in ob/ob mice is improved by TBP-2 deficiencyin vivoandex vivo. Serum insulin concentrations at 11 and 14 weeks aged male (a) and female (b) mice. The median lines are shown in box graphs.n=6–12 per group. Physiological analyses of islet mass (c) and insulin immunostaining of islets (d) in 10 weeks aged mice. Scale bars, 100 μm;n=3 per group. (e) Serum insulin levels during intraperitoneal glucose tolerance tests (IPGTTs). Following an overnight fast, mice were injected with 1 g kg−1glucose, IP (time 0). Serum insulin values were assessed before and at 5, 15, 30 and 45 min into the IPGTT. ob/ob (closed circle,n=6), ob/ob·TBP-2−/− (open circle,n=5). (f–k) Batches of 10 pancreatic islets isolated from WT, TBP-2−/−, ob/ob and ob/ob·TBP-2−/− mice of 10 weeks age were stimulated with 2.8 mM (open bar) or 16.7 mM glucose (closed bar) for 30 min. Insulin secretion (f–h) and ATP contents (i–k) were measured by radioimmunoassay and a luminometer, respectively. WT was compared with TBP-2−/− (f,i) or ob/ob with ob/ob·TBP-2−/− (g,j). Amplification rate of insulin secretion (h) and ATP contents (k) at high (16.7 mM) glucose compared with basal (2.8 mM) glucose stimulation for 30 min. (l) Electron microscopic images of islet sections (×30200; scale bar, 500 nm). Magnified areas of individual β-cell mitochondria. Red arrows highlight individual mitochondria and blue arrows highlight insulin granules. *Swelling and disappearance of cristae structures of mitochondria. Data are presented as mean±s.d. *P<0.05, **P<0.01, ***P<0.001, versus control (t-test). Figure 4: Impairment of glucose-stimulated insulin secretion in ob/ob mice is improved by TBP-2 deficiency in vivo and ex vivo . Serum insulin concentrations at 11 and 14 weeks aged male ( a ) and female ( b ) mice. The median lines are shown in box graphs. n =6–12 per group. Physiological analyses of islet mass ( c ) and insulin immunostaining of islets ( d ) in 10 weeks aged mice. Scale bars, 100 μm; n =3 per group. ( e ) Serum insulin levels during intraperitoneal glucose tolerance tests (IPGTTs). Following an overnight fast, mice were injected with 1 g kg −1 glucose, IP (time 0). Serum insulin values were assessed before and at 5, 15, 30 and 45 min into the IPGTT. ob/ob (closed circle, n =6), ob/ob·TBP-2−/− (open circle, n =5). ( f – k ) Batches of 10 pancreatic islets isolated from WT, TBP-2−/−, ob/ob and ob/ob·TBP-2−/− mice of 10 weeks age were stimulated with 2.8 mM (open bar) or 16.7 mM glucose (closed bar) for 30 min. Insulin secretion ( f – h ) and ATP contents ( i – k ) were measured by radioimmunoassay and a luminometer, respectively. WT was compared with TBP-2−/− ( f , i ) or ob/ob with ob/ob·TBP-2−/− ( g , j ). Amplification rate of insulin secretion ( h ) and ATP contents ( k ) at high (16.7 mM) glucose compared with basal (2.8 mM) glucose stimulation for 30 min. ( l ) Electron microscopic images of islet sections (×30200; scale bar, 500 nm). Magnified areas of individual β-cell mitochondria. Red arrows highlight individual mitochondria and blue arrows highlight insulin granules. *Swelling and disappearance of cristae structures of mitochondria. Data are presented as mean±s.d. * P <0.05, ** P <0.01, *** P <0.001, versus control ( t -test). Full size image TBP-2 suppresses mitochondrial ATP production and GSIS To delineate how TBP-2 deficiency protects against the impaired GSIS in ob/ob islets, we next examined the dose effect of TBP-2 on GSIS in the rat β-cell line INS-1 cells. Silencing of TBP-2 (RNAi1 and RNAi2) enhanced GSIS in INS-1 cells ( Fig. 5a,b,d ). On the contrary, transient TBP-2 overexpression suppressed GSIS ( Fig. 5c,e ). Induction of TBP-2 in cloned INS-1 cells, where TBP-2 expression was doxycycline-off dependent, suppressed GSIS, but not KCl-induced insulin secretion ( Fig. 5f,g ). TBP-2 induction did not cause a significant change in ATP levels at low (2.8 mM) glucose level, but it suppressed ATP levels at high (16.7 mM) glucose in INS-1 cells ( Fig. 5h ). Furthermore, glucose-induced intracellular Ca 2+ elevation, which is the eventual trigger for the exocytosis of insulin granules, was significantly decreased in TBP-2-induced INS-1 cells ( Fig. 5i ). We then analysed mitochondrial membrane potentials ( Δψ m ) in TBP-2-induced INS-1 cells. We showed that Δψ m was significantly reduced in TBP-2-induced INS-1 cells cultured with low (3 mM) and high (20 mM) glucose ( Fig. 5j ) and with 11 mM glucose for 24 h ( Fig. 5k ) using a flowcytometer and fluorescence microscopy, respectively. Cellular ATP is mainly produced by glycolysis and mitochondrial metabolism. In pancreatic β-cells, glycolytic flux regulates glucose metabolism, which has an important role in insulin secretion, and glucokinase is a pace-setting enzyme in glycolysis [31] . Therefore, effects of TBP-2 on glucokinase activity were examined. Glucokinase activity was not affected by dox-off-dependent TBP-2 induction in β-cells ( Fig. 5l ). Furthermore, effects of TBP-2 on insulin secretion stimulated by fuel secretagogues, which bypass glycolysis and are metabolized in mitochondria to generate ATP, were determined using methods previously described [32] . Insulin secretion induced by pyruvate and α-ketoisocaprotate plus monomethyl succinate was also suppressed by TBP-2 overexpression in β-cells ( Fig. 5m ). These results indicate that impaired GSIS by TBP-2 induction is attributable to reduction in mitochondrial metabolism, but not to a decrease in glycolysis. 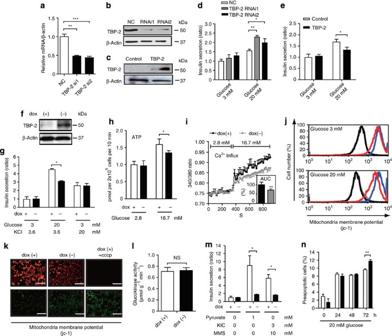Figure 5: TBP-2 suppresses glucose-induced mitochondrial energy production and insulin secretion in β-cells. Transient TBP-2 knockdown by TBP-2 siRNA (RNAi1 and RNAi2) and negative control siRNA (NC) in INS-1 cells. The expression of TBP-2 was determined by qRT–PCR (a) at 48 h after transfection and by immunoblot analysis (b) at 72 h after transfection. (c) Transient TBP-2 overexpression in INS-1 cells after 24 h. The expression of TBP-2 was determined by immunoblot analyses. Augmentation or suppression of GSIS in TBP-2 knockdown (d) or TBP-2 overexpression (e) cells in RPMI cultured medium. Statistic insulin secretion assays were analysed in INS-1 cells. (f) Construction of the doxycycline (dox)-off-dependent TBP-2-overexpressed INS-1 cells. TBP-2 protein was suppressed by 1000 ng ml−1dox and induced by dox removal. Cells were cultured with (+, open bar) or without (−, closed bar) dox for 24 h. INS-1 cells were incubated at low (2.8 or 3 mM) or high (16.7 or 20 mM) glucose and experiments were performed. Suppression of high (20 mM) GSIS (g), high (16.7 mM) glucose-enhanced ATP contents (h) and intracellular Ca2+influx (i) by dox-off TBP-2 overexpression, but not KCl-induced insulin secretion (g). The inset bar graph shows area under the curve levels (%) of intracellular Ca2+levels between 320 and 900 s (i). Decrease of mitochondrial membrane potentials (MMP) in dox-off TBP-2 overexpression in INS-1 cells. MMP of cultured cells in medium containing 3 mM (upper panel) or 20 mM (lower panel) glucose for 24 h was analysed by flow cytometry (j) or in cultured medium by fluorescence microscopy (k) using jc-1 reagent, scale bar is 100 μm. For disruption of MMP, 5 μM carbonyl cyanide m-chlorophenlhydrazone (cccp) reagent was used. Flow cytometer, blue; dox (+), red; dox (−), black; dox (+) + cccp, grey; dox (−) + cccp. (l) Glucokinase (GK) activities in INS-1 cells, NS, nonsignificant. (m) Suppression of pyruvate (sodium pyruvate) or 2-ketoisohexanoic acid (KIC) and methylsaccinic acid (monomethyl succinate)-stimulated insulin secretion by dox-off-dependent TBP-2 overexpression. (n) A flow cytometric analyses with Annexin V-fluorescein isothiocyanate and propidium iodide staining in the dox-off TBP-2-overexpressed INS-1 cells. Preapoptotic cells were calculated from triplicate samples (%). Data are presented as mean±s.d. *P<0.05, **P<0.01, ***P<0.001, versus control (t-test). Figure 5: TBP-2 suppresses glucose-induced mitochondrial energy production and insulin secretion in β-cells. Transient TBP-2 knockdown by TBP-2 siRNA (RNAi1 and RNAi2) and negative control siRNA (NC) in INS-1 cells. The expression of TBP-2 was determined by qRT–PCR ( a ) at 48 h after transfection and by immunoblot analysis ( b ) at 72 h after transfection. ( c ) Transient TBP-2 overexpression in INS-1 cells after 24 h. The expression of TBP-2 was determined by immunoblot analyses. Augmentation or suppression of GSIS in TBP-2 knockdown ( d ) or TBP-2 overexpression ( e ) cells in RPMI cultured medium. Statistic insulin secretion assays were analysed in INS-1 cells. ( f ) Construction of the doxycycline (dox)-off-dependent TBP-2-overexpressed INS-1 cells. TBP-2 protein was suppressed by 1000 ng ml −1 dox and induced by dox removal. Cells were cultured with (+, open bar) or without (−, closed bar) dox for 24 h. INS-1 cells were incubated at low (2.8 or 3 mM) or high (16.7 or 20 mM) glucose and experiments were performed. Suppression of high (20 mM) GSIS ( g ), high (16.7 mM) glucose-enhanced ATP contents ( h ) and intracellular Ca 2+ influx ( i ) by dox-off TBP-2 overexpression, but not KCl-induced insulin secretion ( g ). The inset bar graph shows area under the curve levels (%) of intracellular Ca 2+ levels between 320 and 900 s ( i ). Decrease of mitochondrial membrane potentials (MMP) in dox-off TBP-2 overexpression in INS-1 cells. MMP of cultured cells in medium containing 3 mM (upper panel) or 20 mM (lower panel) glucose for 24 h was analysed by flow cytometry ( j ) or in cultured medium by fluorescence microscopy ( k ) using jc-1 reagent, scale bar is 100 μm. For disruption of MMP, 5 μM carbonyl cyanide m-chlorophenlhydrazone (cccp) reagent was used. Flow cytometer, blue; dox (+), red; dox (−), black; dox (+) + cccp, grey; dox (−) + cccp. ( l ) Glucokinase (GK) activities in INS-1 cells, NS, nonsignificant. ( m ) Suppression of pyruvate (sodium pyruvate) or 2-ketoisohexanoic acid (KIC) and methylsaccinic acid (monomethyl succinate)-stimulated insulin secretion by dox-off-dependent TBP-2 overexpression. ( n ) A flow cytometric analyses with Annexin V-fluorescein isothiocyanate and propidium iodide staining in the dox-off TBP-2-overexpressed INS-1 cells. Preapoptotic cells were calculated from triplicate samples (%). Data are presented as mean±s.d. * P <0.05, ** P <0.01, *** P <0.001, versus control ( t -test). Full size image TBP-2 has been reported to enhance apoptosis in pancreatic β-cells and other cells [21] . TBP-2 induction did not increase apoptosis in 48 h, but apoptosis was slightly increased on 72 h after high (20 mM) glucose treatment ( Fig. 5n ). β-Cell apoptosis was not changed significantly between ob/ob and ob/ob TBP-2−/− mice generated in a C57BL/6J background at 10 weeks of age ( Supplementary Figs S3a,b and S4a ), whereas TBP-2 deficiency suppressed β-cell apoptosis at age 36 weeks in C57BL/6J background mice ( Supplementary Fig. S4b,c ).These results suggest that TBP-2 negatively regulates GSIS by suppressing glucose-induced mitochondrial ATP production in INS-1 cells and islets before causing apoptosis. Treatment with reactive oxygen species scavengers (vitamins C+E) scarcely recovered the insulin secretion suppressed by TBP-2 overexpression in INS-1 cells ( Supplementary Fig. S5 ), suggesting that mitochondrial dysfunction caused by TBP-2 is not mainly attributed to an increase in reactive oxygen species by reducing the scavenger effect of thioredoxin. TBP-2 enhances UCP-2 transcriptional activity Impairment in mitochondria ATP production often occurs with uncoupling [24] . Mitochondrial UCP-2 is a key regulator of ATP production and insulin secretion in pancreatic β-cells, and UCP-2 deficiency has been shown to improve GSIS and glucose-induced ATP production in ob/ob mice [24] . Thus, we measured UCP-2 mRNA in TBP-2-overexpressed INS-1 cells. Strikingly, there was a significant increase in UCP-2 mRNA levels in the TBP-2-induced cells ( Fig. 6a ). Furthermore, TBP-2 induction also increased UCP-2 protein levels in the mitochondria of INS-1 cells ( Fig. 6b ). UCP-2 expression is known to be upregulated by the increase in activity of transcriptional co-activators; e.g., PPARγ co-activator-1α (PGC-1α) [33] . TBP-2 is also induced by PGC-1α overexpression in INS-1 cells ( Fig. 6c ). We examined the effect of TBP-2 overexpression on activity of UCP-2 -86 promoter, containing Sp1, SRE and double E-box elements, the essential elements for a response to fatty acids and PGC-1α [33] , [34] . TBP-2 enhanced UCP-2 transcriptional activity through this -86 promoter region and the PGC-1α-induced activation was also augmented by TBP-2 expression ( Fig. 6d ), suggesting that TBP-2 enhances UCP-2 transcriptional activity and expression in INS-1 cells. To investigate how TBP-2 regulates UCP-2 transcriptional activity, we tested whether TBP-2 affects PGC-1α protein levels. Dox-off-dependent TBP-2 overexpression did not change PGC-1α protein levels ( Supplementary Fig. S6 ). Next, we used chromatin immunoprecipitations (ChIPs) to investigate whether TBP-2 expression influences PGC-1α binding efficiency to the UCP-2 promoter region. Sheared chromatin was collected from INS-1 cells treated with or without doxycycline, and then immunoprecipitated with anti-RNA polymerase II or control-mouse immunoglobulin G or anti-PGC-1α antibody. PCR was performed with primers flanking the SP1, SRE and E-boxes region of UCP-2 (UCP-2 -86). PGC-1α was recruited to the UCP-2 -86 promoter region and dox-off-dependent TBP-2 overexpression enhanced PGC-1α binding efficiency to the region ( Fig. 6e,f ). These results indicate that TBP-2 facilitates PGC-1α recruitment in the UCP-2 promoter region, enhancing UCP-2 transcriptional activity in INS-1 cells. Next, we tested whether TBP-2-dependent UCP-2 expression is critical for aggravated GSIS using UCP-2 knockdown in dox-off-dependent TBP-2-overexpressing INS-1 cells. UCP-2 knockdown reversed suppression of GSIS by TBP-2 induction ( Fig. 6g and Supplementary Fig. S7 ), suggesting that TBP-2-induced suppression of GSIS is mainly through UCP-2 expression. 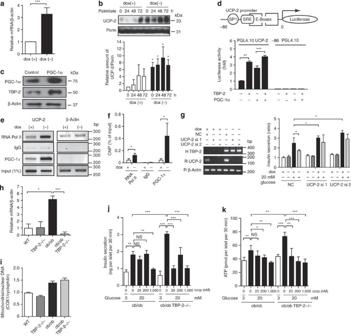Figure 6: TBP-2 enhances UCP-2 transcriptional activity. (a) Quantitative RT–PCR (qRT–PCR) analyses of UCP-2 mRNA expression in dox-off-dependent TBP-2-overexpressed INS-1 cells with or without dox. (b) Immuno blotting to determine UCP-2 expression in mitochondria in dox-off TBP-2 overexpression in INS-1 cells with or without palmitate (300 μM) for the indicated time. Densitometric quantification of the UCP-2/Porin ratio in mitochondria of INS-1 cells is shown in a bar graph. (c) Immuno blotting analyses to detect expression of PGC-1α, TBP-2 and β-actin in INS-1 cells, transiently transfected with PGC-1α plasmid for 24 h. (d) INS-1 cells were transfected with PGL4.10 UCP-2 -86 or PGL4.10-luciferase reporter plasmid and each expression plasmid for PGC-1α and TBP-2, as indicated. Luciferase reporter activity was normalized byRenillaluciferase activity. (e) ChIP assay of PGC-1α protein binding to endogenous UCP-2 promoter. Chromatin extracts from INS-1 cells in dox-off-dependent TBP-2-overexpressed INS-1 cells with or without dox were precipitated in the presence of control-mouse IgG, anti-RNA polymerase II (RNA pol II) or anti-PGC-1α antibody. Primers for PCR are rat UCP-2 promoter region primers and rat β-actin primers. (f) qRT–PCR analyses for ChIP were performed. (g) Insulin secretion in dox-off-dependent TBP-2 overexpressing INS-1 cells with or without dox and knockdown of UCP-2 (si1 and si2). The left panel shows RT–PCR analysis of humanTBP-2expression (H TBP-2) to confirm the effect of dox, ratUCP-2expression (R UCP-2) to confirm the knockdown effect, and rat β-actin(R β-actin). (h) qRT–PCR analyses of UCP-2 mRNA in isolated pancreatic islets of WT, TBP-2−/−, ob/ob and ob/ob·TBP-2−/− mice. (i) qRT–PCR was used to determine mitochondria content by measuring the expression of mitochondrial gene (COX I)/nuclear gene (cyclophilin) ratios. (j,k) Effect of cccp treatment for 30 min on insulin secretion (j, ng per islet per 30 min) and ATP levels (k, pmol per islet per 30 min) in ob/ob and ob/ob TBP-2−/− islets. Data are presented as mean±s.d. *P<0.05, **P<0.01, ***P<0.001, versus control (t-test). Furthermore, the expression level of UCP-2 mRNA was enhanced in islets of ob/ob mice, whereas TBP-2 deficiency dramatically reduced it in ob/ob islets ( Fig 6h ). Mitochondrial mass, determined as mitochondrial coding gene (mtDNA)/nuclear coding gene (COX I) expression ratio in pancreatic islets, was not affected by TBP-2 deficiency ( Fig. 6i ). Next, we examined the effect of the mitochondrial uncoupler carbonyl cyanide m-chlorophenyl-hydrazone (cccp) on GSIS in Tet-TBP-2 INS-1 cells with or without doxycycline and in TBP-2 deficient ob/ob islets. Uncoupling by cccp decreased the GSIS at the concentration 25–1,000 nM ( Supplementary Fig. S8a ). This result suggests that mitochondria metabolism is responsible for GSIS in β-cells and is tightly regulated by uncoupling. In dox-off tet-TBP-2 INS-1 cells, TBP-2 overexpression suppressed the GSIS equivalent to the level elicited by 25 nM cccp ( Supplementary Fig. S8b ). More importantly, cccp had a larger effect on GSIS and glucose-induced ATP production in TBP-2-deficient ob/ob islets compared with ob/ob islets ( Fig. 6j,k ). These results suggest that TBP-2-dependent regulation of GSIS is mainly achieved through mitochondrial uncoupling and metabolism. Figure 6: TBP-2 enhances UCP-2 transcriptional activity. ( a ) Quantitative RT–PCR (qRT–PCR) analyses of UCP-2 mRNA expression in dox-off-dependent TBP-2-overexpressed INS-1 cells with or without dox. ( b ) Immuno blotting to determine UCP-2 expression in mitochondria in dox-off TBP-2 overexpression in INS-1 cells with or without palmitate (300 μM) for the indicated time. Densitometric quantification of the UCP-2/Porin ratio in mitochondria of INS-1 cells is shown in a bar graph. ( c ) Immuno blotting analyses to detect expression of PGC-1α, TBP-2 and β-actin in INS-1 cells, transiently transfected with PGC-1α plasmid for 24 h. ( d ) INS-1 cells were transfected with PGL4.10 UCP-2 -86 or PGL4.10-luciferase reporter plasmid and each expression plasmid for PGC-1α and TBP-2, as indicated. Luciferase reporter activity was normalized by Renilla luciferase activity. ( e ) ChIP assay of PGC-1α protein binding to endogenous UCP-2 promoter. Chromatin extracts from INS-1 cells in dox-off-dependent TBP-2-overexpressed INS-1 cells with or without dox were precipitated in the presence of control-mouse IgG, anti-RNA polymerase II (RNA pol II) or anti-PGC-1α antibody. Primers for PCR are rat UCP-2 promoter region primers and rat β-actin primers. ( f ) qRT–PCR analyses for ChIP were performed. ( g ) Insulin secretion in dox-off-dependent TBP-2 overexpressing INS-1 cells with or without dox and knockdown of UCP-2 (si1 and si2). The left panel shows RT–PCR analysis of human TBP-2 expression (H TBP-2) to confirm the effect of dox, rat UCP-2 expression (R UCP-2) to confirm the knockdown effect, and rat β- actin (R β-actin). ( h ) qRT–PCR analyses of UCP-2 mRNA in isolated pancreatic islets of WT, TBP-2−/−, ob/ob and ob/ob·TBP-2−/− mice. ( i ) qRT–PCR was used to determine mitochondria content by measuring the expression of mitochondrial gene (COX I)/nuclear gene (cyclophilin) ratios. ( j , k ) Effect of cccp treatment for 30 min on insulin secretion ( j , ng per islet per 30 min) and ATP levels ( k , pmol per islet per 30 min) in ob/ob and ob/ob TBP-2−/− islets. Data are presented as mean±s.d. * P <0.05, ** P <0.01, *** P <0.001, versus control ( t -test). Full size image These results suggest that TBP-2 does not affect mitochondrial biogenesis but enhances UCP-2 transcriptional activity through the PGC-1α-dependent pathway, and the induction of the TBP-2-UCP-2 axis causes the defect of GSIS in ob/ob mice. Mybbp1a is a novel candidate binding protein for TBP-2 To obtain further insight on how TBP-2 regulates gene expression in β-cells, we purified the TBP-2 protein complex using tosyl (p-toluene sulfonyl)-activated magnetic beads (Ts beads). His-tagged-TBP-2 protein was conjugated to the beads and incubated with nuclear extract of INS-1 cells. After washing, the eluate fractions were subjected to SDS gel electrophoresis and silver staining ( Fig. 7a ). The specific bands on silver staining were subjected to proteolytic digestion and mass spectrometry. Mybbp1a (p160), Mybbp1a (p140), GCN and NonO/p54nrb homologue were identified ( Fig. 7b and Supplementary Table S3 ). Intriguingly, Mybbp1a is reported to inhibit PGC-1α function and transcription of PGC-1α target genes [35] . Therefore, we examined the interaction between TBP-2 and Mybbp1a. We showed that Mybbp1a is detected in elution samples from TBP-2 protein beads by anti-Mybbp1a antibody ( Fig. 7c ). To determine whether TBP-2 and Mybbp1a interact directly in vivo , we performed co-immunoprecipitation using FLAG-HA-tagged Mybbp1a and Myc-tagged TBP-2 expression vectors. Myc-tagged TBP-2 was co-immunoprecipitated with FLAG-HA-tagged Mybbp1a in HEK293 cells ( Fig. 7d ). Finally, we examined whether Mybbp1a regulates UCP-2 transcriptional activity. Mybbp1a suppressed PGC-1α-dependent UCP-2 transcriptional activity and the suppression was reversed by TBP-2 co-expression ( Fig. 7e ). These results provide a model that TBP-2 suppresses Mybbp1a function possibly through protein–protein interaction, leading to the activation of PGC-1α-dependent UCP-2 transcription ( Fig. 7f ). 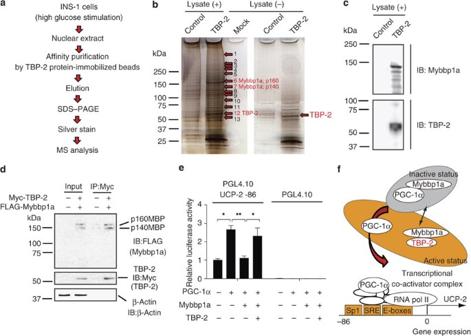Figure 7: Mybbp1a was identified as a novel candidate binding protein for TBP-2. (a) Purification scheme for the TBP-2 containing protein complex in β-cell nuclear extracts. TBP-2 binding proteins were purified from INS-1 nuclear extracts by using TBP-2 protein-immobilized (TBP-2) or control beads. (b) Identification of the TBP-2 complex. Silver staining was performed. Numbers indicate individual candidate proteins interacting with TBP-2. (c) Eluted proteins were analysed by immuno blotting (IB) for Mybbp1a and TBP-2 antibody. (d) Co-immunoprecipitation analyses. Input (left, 5% lysate) and anti-Myc immunoprecipitates (right, IP:Myc) from HEK293 cells transfected with pCMV-tag2A and pCMV-tag3B vector (−) or FLAG-HA-Mybbp1a and Myc-TBP-2 vector (+) were analysed by immunoblotting (IB) with antibodies to FLAG, Myc and β-actin. The positions for Mybbp1a (p160; p160MBP) and Mybbp1a (p140; p140MBP) (upper), TBP-2 (middle) and β-actin (lower) are shown. (e) Luciferase activity of the UCP-2 -86 enhancer region. INS-1 cells were transfected with PGL4.10 UCP-2 -86 or PGL4.10-luciferase reporter plasmid and each expression plasmid for PGC-1α, Mybbp1a and TBP-2, as indicated. Luciferase reporter activity was normalized byRenillaluciferase activity. (f) A schematic model of TBP-2 function in β-cells. Mybbp1a binds PGC-1α (inactive form) and inhibits UCP-2 transcriptional activity. Induced TBP-2 interacts with Mybbp1a and releases PGC-1α from Mybbp1a, facilitating PGC-1α recruitment on the UCP-2 promoter region. Data are presented as mean±s.d. *P<0.05, **P<0.01, versus control (t-test). Figure 7: Mybbp1a was identified as a novel candidate binding protein for TBP-2. ( a ) Purification scheme for the TBP-2 containing protein complex in β-cell nuclear extracts. TBP-2 binding proteins were purified from INS-1 nuclear extracts by using TBP-2 protein-immobilized (TBP-2) or control beads. ( b ) Identification of the TBP-2 complex. Silver staining was performed. Numbers indicate individual candidate proteins interacting with TBP-2. ( c ) Eluted proteins were analysed by immuno blotting (IB) for Mybbp1a and TBP-2 antibody. ( d ) Co-immunoprecipitation analyses. Input (left, 5% lysate) and anti-Myc immunoprecipitates (right, IP:Myc) from HEK293 cells transfected with pCMV-tag2A and pCMV-tag3B vector (−) or FLAG-HA-Mybbp1a and Myc-TBP-2 vector (+) were analysed by immunoblotting (IB) with antibodies to FLAG, Myc and β-actin. The positions for Mybbp1a (p160; p160MBP) and Mybbp1a (p140; p140MBP) (upper), TBP-2 (middle) and β-actin (lower) are shown. ( e ) Luciferase activity of the UCP-2 -86 enhancer region. INS-1 cells were transfected with PGL4.10 UCP-2 -86 or PGL4.10-luciferase reporter plasmid and each expression plasmid for PGC-1α, Mybbp1a and TBP-2, as indicated. Luciferase reporter activity was normalized by Renilla luciferase activity. ( f ) A schematic model of TBP-2 function in β-cells. Mybbp1a binds PGC-1α (inactive form) and inhibits UCP-2 transcriptional activity. Induced TBP-2 interacts with Mybbp1a and releases PGC-1α from Mybbp1a, facilitating PGC-1α recruitment on the UCP-2 promoter region. Data are presented as mean±s.d. * P <0.05, ** P <0.01, versus control ( t -test). Full size image In this study, we demonstrated that disruption of TBP-2 expression augments both insulin sensitivity and secretion, resulting in the amelioration of glucose intolerance in a diabetic mice model where TBP-2 expression is increased. The mechanism by which TBP-2 is increased in several tissues and pancreatic islets of ob/ob mice is presently unknown. It is possible that high blood glucose or obese-induced adipocytokines enhance TBP-2 expression, as TBP-2 is upregulated by several stimulations and stresses [36] , [37] . Several reports have shown that TBP-2 expression is regulated by mitochondrial metabolism and glycolysis through the transcription factor MondoA [38] , [39] , [40] , [41] . These reports indicate that TBP-2 expression is tightly regulated in response to changes in energy status. TBP-2 deficiency in ob/ob mice improved hyperglycaemia, glucose intolerance and insulin resistance without amelioration of obesity ( Fig. 1e–m ). A previous study showed that HcB-19 mice crossed with ob/ob mice improved glucose tolerance [21] . Other studies showed that silencing of TBP-2 expression enhanced glucose uptake in adipocytes and human skeletal myocytes, whereas TBP-2 overexpression inhibited glucose uptake [19] . Entire or muscle-specific TBP-2−/− mice showed enhanced glucose uptake in the skeletal muscle and adipose with a high-fat diet [23] , [42] . The current study is consistent with these previous reports. The restoration of glucose tolerance in ob/ob·TBP-2−/− mice could not be explained by changes in energy balance or hormonal level of adipocytokines, such as adiponectin, free fatty acids and MCP-1. Insulin resistance in skeletal muscle and liver is mainly caused by inactivation of insulin/Akt signalling [1] . We showed that TBP-2 deficiency in ob/ob mice improved Akt signalling in muscle but not liver ( Fig. 2k–p ). Moreover, IRS-1 gene and several insulin signalling genes were upregulated in skeletal muscle by TBP-2 deficiency both in WT and ob/ob mice ( Fig. 3a and Supplementary Table S2 ). IRS-1 protein levels were downregulated in the skeletal muscle of ob/ob mice compared with that of WT mice, while IRS-1 protein levels were also upregulated by TBP-2 deficiency in both WT and ob/ob mice ( Fig. 3b ). As IRS-1 has a pivotal role in insulin sensitivity in muscle [27] , TBP-2 regulates insulin signalling possibly through the regulation of IRS-1 gene expression in muscle. Interestingly, TBP-2 deficiency did not change IRS-2 gene expression, which is known as a main regulator of liver insulin sensitivity [43] in skeletal muscle ( Fig. 3a ). These results suggest that TBP-2 regulates IRS-1-related insulin sensitivity in skeletal muscle, but not IRS-2-related insulin sensitivity in liver. The molecular mechanism of how TBP-2 regulates the expression of IRS-1 and insulin signalling genes in skeletal muscle is now under investigation. We also found that gene expression of PPARs and their target genes, such as PPARγ , PPARα , Acaca , Fabp3 , Scd1 and Pdk4 , are enhanced by TBP-2 deficiency in skeletal muscle ( Supplementary Fig. S2 ), similar to previous reports in the liver and adipose tissue of TBP-2−/− mice [16] , [42] . As PPAR signalling augments insulin sensitivity [44] , it may also be involved in enhanced insulin sensitivity by TBP-2 deficiency. The GSIS was significantly impaired in ob/ob islets, whereas insulin secretion from ob/ob·TBP-2−/− islets was restored in vivo and ex vivo , suggesting that the ablation of TBP-2 in pancreatic islets of ob/ob mice augments GSIS. Our results indicate that upregulation of TBP-2 suppresses GSIS by reducing ATP production in pancreatic β-cells. Meanwhile, glycolytic activity was not changed by TBP-2 overexpression ( Fig. 5l ) in β-cell lines. Recently, several groups have shown that TBP-2 regulates β-cell mass and β-cell apoptosis in C3H/He background mice and INS-1 cells [21] , [22] , [45] , [46] . Our results also support these previous studies. TBP-2 deficiency suppressed β-cell apoptosis at age 36 weeks in C57BL/6J background mice ( Supplementary Fig. S4b,c ). In contrast, while β-cell apoptosis was not changed significantly between ob/ob and ob/ob·TBP-2−/− mice generated in C57BL/6J background mice at 10 weeks age ( Supplementary Figs S3a,b and S4a,c ), TBP-2 deficiency improved GSIS in ob/ob mice at age 10–14 weeks. Taken together, improvement of GSIS by TBP-2 depletion in vivo was attributable to functional amelioration of β-cells but not to an increase in β-cell mass, at least, in mice of this age. Moreover, impaired GSIS without reduction in β-cell mass preceded significant detection of apoptosis in islets in ob/ob mice, which supports the pathogenic importance of functional impairment of β-cells. Thus, TBP-2 seems to regulate not only β-cell apoptosis but also β-cell energy metabolism in the diabetic condition. Impairment of GSIS in ob/ob mice was improved by TBP-2 deficiency. This phenotype resembles ob/ob mice lacking UCP-2, which is a negative regulator of GSIS [24] . We showed that TBP-2 deficiency cancelled upregulation of UCP-2 gene expression in ob/ob islets ( Fig. 6h ). Therefore, UCP-2 regulation by TBP-2 seems to be important in the development of the diabetic phenotype in ob/ob mice. UCP-2 knockdown recovered the TBP-2-dependent impairment in GSIS ( Fig 6g ). Furthermore, the mitochondrial uncoupling reagent cccp had a greater effect on GSIS and glucose-induced ATP production in TBP-2-deficient ob/ob islets compared with those in ob/ob islets ( Fig. 6j,k ). These results suggest that TBP-2-dependent regulation of GSIS is mainly due to mitochondrial uncoupling derived from UCP-2 expression. The results from a ChIP assay indicated that TBP-2 regulates UCP-2 expression by facilitating PGC-1α recruitment to the UCP-2 promoter region. Furthermore, we identified Mybbp1a as a novel binding protein of TBP-2. Mybbp1a is reported to inhibit PGC-1α function and transcription of PGC-1α target genes through direct protein–protein interaction [35] . Indeed, Mybbp1a overexpression suppressed PGC-1α-dependent UCP-2 transcriptional activity ( Fig. 7e ), and TBP-2 overexpression hampered the effect of Mybbp1a on PGC-1α-dependent UCP-2 promoter activity in INS-1 cells ( Fig. 7e ). These results suggest a model that TBP-2 regulates UCP-2 expression through Mybbp1a and PGC-1α pathway ( Fig. 7f ). Recently, it has been reported that α-arrestin family proteins are considered to act as adaptor protein for the E3-ubiquitin ligases in the yeast system [47] and TBP-2 interacts with WW domain of HECT domain containing E3-ubiquitin ligases through the PPxY motif of TBP-2 [12] . These reports provide a hypothesis that TBP-2 negatively regulates Mybbp1a by protein degradation through E3-ubiquitin ligases. This possibility should be further investigated. In this study, we demonstrated that ablation of TBP-2 expression augments both insulin sensitivities by enhancing IRS-1/Akt signalling in skeletal muscle and GSIS by suppressing UCP-2 transcription and maintaining mitochondrial function in pancreatic β-cells, resulting in the amelioration of glucose intolerance and hyperglycaemia. 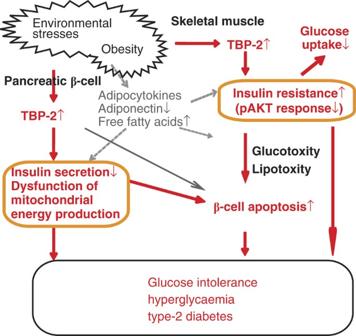Figure 8: A model for metabolic function of TBP-2 in diabetes. Role of TBP-2 in promoting obesity-induced type 2 diabetes. Environmental stresses including obesity cause upregulation of TBP-2. Sustained expression of TBP-2 may impair mitochondrial function and insulin secretion in β-cells and aggravate insulin resistance in skeletal muscle. Augmented expression of TBP-2 may also result in β-cell apoptosis. These changes lead to glucose intolerance and hyperglycaemia and obese-induced type 2 diabetes. The proposed mechanism for this effect is summarized in Figure 8 and Supplementary Figure S9 . These findings raise the possibility that the inhibition of either TBP-2 activity or expression may be a novel therapeutic approach for type 2 diabetes. Figure 8: A model for metabolic function of TBP-2 in diabetes. Role of TBP-2 in promoting obesity-induced type 2 diabetes. Environmental stresses including obesity cause upregulation of TBP-2. Sustained expression of TBP-2 may impair mitochondrial function and insulin secretion in β-cells and aggravate insulin resistance in skeletal muscle. Augmented expression of TBP-2 may also result in β-cell apoptosis. These changes lead to glucose intolerance and hyperglycaemia and obese-induced type 2 diabetes. Full size image Animal experiments TBP-2-knockout mice were generated as described previously [17] . Mice were backcrossed for at least 11 generations with a C57B/6 genetic background. Animals were maintained in a specific pathogen-free animal facility on a 12-h light–dark cycle at an ambient temperature of 21 °C. They were given free access to water and food. Age- and sex-matched mice were used for all animal experiments. All procedures involving animals were performed in accordance with protocols approved by the Animal Care and Research Advisory Committee of the Institute for Virus Research at Kyoto University. Generation of TBP-2-deficient ob/ob mice C57BL6 ob/+ were purchased from the Jackson Laboratory. To generate ob/ob·TBP-2−/− mice, TBP-2−/− mice were crossed with ob/+ mice creating compound heterozygotes, ob/OB·TBP-2+/−. In the second cross, compound heterozygotes were crossed to generate the following animals of which both males and females were collected and studied further: WT mice (+/+ at both ob and TBP-2 loci), ob/ob mice (ob/ob at the ob locus and +/+ at the TBP-2 locus), TBP-2−/− mice (+/+ at the ob locus and −/− at the TBP-2 locus) and ob/ob·TBP-2−/− mice (ob/ob at the ob locus and −/− at the TBP-2 locus). The ob allele was genotyped as previously described [48] . Intraperitoneal glucose or ITTs For the intraperitoneal (IP) glucose tolerance test, following an overnight fast, ob/ob and ob/ob·TBP-2−/− mice were injected with 0.5 g kg −1 or 1 g kg −1 glucose. Blood glucose values were assessed before and at 15, 30, 60 and 120 min after the IP administration of glucose using glucose PILOT. Serum insulin values were assessed before and at 5, 15, 30 and 45 min after the IP administration of glucose using an Insulin ELISA kit. For the IP ITTs, mice were fasted for 6 h and then injected with 1 U kg −1 insulin. Cell culture and transfection INS-1 cells were cultured at 37 °C with 5% CO 2 in air in RPMI1640 (Sigma-Aldrich), supplemented with 10% (v/v) fetal bovine serum, 1% (v/v) penicillin/streptomycin antibiotics, 10 mM HEPES, 2 mM L -glutamine, 1 mM sodium pyruvate and 50 μM β-mercaptoethanol (RPMI for INS-1 medium). INS-1 cells were transfected with TBP-2 small interfering RNA (siRNA) or negative control siRNA (Qiagen) for 72 h or with pCMV-Tag2B-TBP-2 or control pCMV-Tag2B (Stratagene) plasmid for 24 h and cultured with RPMI1640 for INS-1 medium. Isolated pancreatic islet studies Pancreatic islets were isolated from mice according to a method used for rats [49] . Generation of INS-1 cells with inducible TBP-2 expression Stable INS-1 cells, which carry the reverse tetracycline/doxycycline-dependent transactivator pTRE2 (pTet-Off, Clontech), were prepared. After selection with 500 μg ml −1 G418, resistant colonies were isolated with limiting dilution methods in 96-well plates. One clonal line that exhibited very high tetracycline-off-inducible luciferase activity and undetectable basal luciferase activity was chosen and used for a second round of transfection with the TBP-2 expression plasmid (pTRE2 pur-TBP-2-FLAG). After selection with 500 ng ml −1 puromycin and doxycycline-off-induced TBP-2 expression, clones were isolated. Insulin secretion assay using INS-1 cells INS-1 cells were transfected with TBP-2 siRNA (Rn_Txnip_1 and 5) or UCP-2 siRNA (Rn_UCP-2_5 and 6) or negative control siRNA (purchased from Qiagen) for 72 h, or with pCMV-Tag2A-TBP-2 or control pCMV-Tag2A (Stratagene) plasmid for 24 h. Then, the cells were cultured in Krebs Ringer bicarbonate buffer (KRBB) (as mentioned below) or RPMI1640 for INS-1 medium with 2.8 mM (5 mM) or 16.7 mM (20 mM) glucose containing RPMI medium and the supernatant was collected 30 min after the addition of glucose. Insulin concentration was measured by an Insulin ELISA kit. Similar analyses were performed in Tet-TBP-2 INS-1 cells pretreated with or without doxycycline for 24 to 48 h. One mM pyruvate (sodium pyruvate, Nacalai Tesque) or 3 mM α-ketoisocaprotate (2-ketoisohexanoic acid, Nacalai Tesque) and 10 mM monomethyl succinate (methylsuccinic acid sodium salt, Sigma-Aldrich)-stimulated insulin secretion assays were performed in Tet-TBP-2 INS-1 cells. Insulin secretion assay using primary mouse pancreatic islet Insulin release from intact islets was monitored using batch incubation methods [50] . Isolated pancreatic islets were precultured at 37 °C for 30 min with gentle swinging (50 times per min) in KRBB containing 129.4 mM NaCl, 3.7 mM KCl, 2.7 mM CaCl 2 , 1.3 mM KH 2 PO 4 , 1.3 mM MgSO 4 , 24.8 mM NaHCO 3 (equilibrated with 5% CO 2 , 95% O 2 , pH 7.4), and 0.2 % (vol/vol) bovine serum albumin (fraction V) with 2.8 mM glucose. Next, the pancreatic islets were incubated for 30 min in KRBB buffer with glucose 2.8 or 16.7 mM to determine insulin secretion levels. At the end of the incubation period, islets were pelleted by centrifugation, and aliquots of the buffer were sampled. The amount of immunoreactive insulin was determined by radioimmunoassay, using rat insulin as standard. ATP contents assay INS-1 cells (2.0×10 5 cells per 24-well plate) or isolated pancreatic islets were precultured in KRBB buffer with 2.8 mM glucose for 2 h or 30 min, and were batch incubated for 10 or 30 min in KRBB with 2.8 or 16.7 mM glucose, respectively. After immediate addition of HClO 4 , cells were sonicated in ice-cold water for 10 min, and centrifuged. Part of the supernatant fraction was mixed with HEPES and Na 2 CO 3 and the ATP content in the cells was determined by luminometer as previously described [50] . Intracellular Ca 2+ + assay INS-1 cells were precultured for 2 h in KRBB with 2.8 mM glucose and then cells were loaded with 5 μM Fura-PE3 AM in KRBB containing 2.8 mM glucose and 0.2% bovine serum albumin at 37 °C for 20 min. Intracellular Ca 2+ concentration was measured by the ratio of emission fluorescence of 510 nm by excitation at 340 and 380 nm as previously described [50] . Measurement of mitochondrial membrane potentials Briefly, INS-1 cells were preincubated in KRBB with 3 and 20 mM glucose or in cultured medium for 24 h, and the cells were resuspended in 0.5 ml of ice-cold PBS, then cultured with 10 nM jc-1 (Sigma-Aldrich, J-4519) for 15 min in 5% CO 2 at 37 °C with or without 5 μM cccp, a protonophore that completely dissipated Δψ , and was analysed by flow cytometry (FACSCanto II, BD Bioscience) or fluorescence microscopy (Biozero, Keyence). The greater the mitochondrial membrane potential, the more jc-1 aggregates form that have a red fluorescent emission signal, as opposed to the jc-1 monomer that fluorescences green. Data acquisition and analysis were performed using Cell Quest Software. Luciferase reporter assays INS-1 cells were transiently transfected with pGL4.10 luc2 vectors containing UCP-2 -86 enhancer region (5′-GGCTCCGCCTCGTCACGCCACGCCCCGACCACGCCCTCTAGA-3′) or pGL4.10 luc2 vectors, with the pCMV-PGC-1α, pCMV-Tag2A-TBP-2 and FLAG-HA-p160 MBP plasmids. FLAG-HA-p160 MBP was kindly provided by Dr Shunsuke Ishii. As a control, the total amount of vectors for transfection was adjusted by the amount of the pCMV-Tag2A vector. After 18 h of transfection, luciferase activity was quantified using the luciferase assay system (Promega). pRL-TK (Promega) was used to monitor Renilla luciferase gene expression as a control for the efficiency of transfection. Cell culture of primary MEFs Primary MEFs were derived from 13.5-day-old embryos from TBP-2+/− mice, and then the MEFs were genotyped to obtain TBP-2−/− and TBP-2+/+ MEFs. Cells were maintained in DMEM with 10% fetal calf serum, 1% penicillin and 0.5% L -glutamine. TBP-2 mRNA expression was confirmed by semiquantitative RT–PCR analysis. Primer sequences are listed in Supplementary Table S4 . Quantitative (semiquantitative) RT–PCR analysis Total RNA was extracted from INS-1 cells or handpicked freshly isolated islets using TRIzol reagent (Invitrogen). Reverse transcription was performed with SuperScript III (Invitrogen) or PrimeScript RT (TAKARA). Real-time RT–PCR was performed using SYBR Premix Ex Tag II(TAKARA). The internal control used was β-actin. PCR analyses were carried out using the oligonucleotide primers listed in Supplementary Table S4 . Chromatin immunoprecipitation Chromatin was prepared from Tet-TBP-2 INS-1 cells treated with or without doxycycline. Briefly, 5×10 6 cells were crosslinked with 1% formaldehyde for 10 min, followed by the addition of glycine at 125 mM. Chromatin was sheared by enzymes (CHIP IT Express Kit, Active Motif). Chromatin was immunoprecipitated with 2 μg anti-RNA polymerase II (Active Motif), control-mouse immunoglobulin G (Active Motif) or anti-PGC-1α antibodies (Santa Cruz). GATCTGAGACAGGGAGACTCTAGG and GGAGAATACACAGGAGAACACAGG primers were used to amplify the UCP-2 SP1, SRE, E-boxes region. Rat β-actin enhancer primers (Active Motif) were used as control. PCR was carried out with one cycle at 95 °C for 2 min; 36 cycles at 94 °C for 10 s, 60 °C for 30 s, 68 °C for 1 min; and one cycle at 68 °C for 5 min. Co-immunoprecipitation To investigate interactions between TBP-2 and Mybbp1a in vivo , Myc-TBP-2 and FLAG-HA-Mybbp1a or pCMV-tag3B and pCMV-tag2A (as control) were co-expressed in HEK293 cells. Cells were lysed in lysis buffer (CellLytic M Cell Lysis Reagent, Sigma-Aldrich), and insoluble materials were precipitated by centrifugation at 15,000× g for 15 min. The resulting supernatants were incubated with anti-Myc agarose beads (MBL), and bound material was eluted with Myc-peptide (500 μg ml −1 , MBL). Protein–protein interaction was assessed by immunoblotting using anti-FLAG antibody (Sigma-Aldrich) or anti-Myc antibody (Sigma-Aldrich). Statistical method Results were expressed as the mean±s.d. Statistical comparisons were made using Student's t -test. A statistically significant difference was defined as * P <0.05, ** P <0.01, *** P <0.001. How to cite this article: Yoshihara, E. et al . Disruption of TBP-2 ameliorates insulin sensitivity and secretion without affecting obesity. Nat. Commun. 1:127 doi: 10.1038/ncomms1127 (2010).